Tumour suppressor TRIM33 targets nuclear β-catenin degradation Aberrant activation of β-catenin in the nucleus has been implicated in a variety of human cancers, but the fate of nuclear β-catenin is unknown. Here we demonstrate that the tripartite motif-containing protein 33 (TRIM33), acting as an E3 ubiquitin ligase, reduces the abundance of nuclear β-catenin protein. TRIM33-mediated β-catenin is destabilized and is GSK-3β or β-TrCP independent. TRIM33 interacts with and ubiquitylates nuclear β-catenin. Moreover, protein kinase Cδ, which directly phosphorylates β-catenin at Ser715, is required for the TRIM33–β-catenin interaction. The function of TRIM33 in suppressing tumour cell proliferation and brain tumour development depends on TRIM33-promoted β-catenin degradation. In human glioblastoma specimens, endogenous TRIM33 levels are inversely correlated with β-catenin. In summary, our findings identify TRIM33 as a tumour suppressor that can abolish tumour cell proliferation and tumorigenesis by degrading nuclear β-catenin. This work suggests a new therapeutic strategy against human cancers caused by aberrant activation of β-catenin. The Wnt/β-catenin pathway, which is often referred to as the canonical Wnt pathway, is a highly conserved signalling cascade that employs β-catenin as a transcriptional coactivator [1] . In the absence of Wnt stimulation, cytoplasmic β-catenin is constitutively targeted for degradation by two multidomain scaffolding proteins, Axin and adenomatous polyposis coli (APC), which facilitate the amino-terminal phosphorylation of β-catenin via the kinases glycogen synthase kinase (GSK)-3 and casein kinase Iα [2] , [3] . Phosphorylated β-catenin is recognized by the E3 ubiquitin ligase β-transducin repeat-containing protein (β-TrCP) and is thus ubiquitinated and degraded by the proteasome. Upon Wnt stimulation, a Wnt ligand binds to the seven-pass transmembrane receptor Frizzled and the single-pass low-density lipoprotein receptor-related protein 5 or 6. This trimeric complex recruits the proteins Dishevelled and Axin, resulting in inhibition of β-catenin phosphorylation and the ensuing β-catenin stabilization [2] , [3] . Stabilized β-catenin then enters the nucleus and activates transcription of downstream target genes via the T-cell factor/lymphoid enhancer-binding factor family of transcription factors [4] . Because β-catenin also regulates cell–cell adhesion by interacting with cadherin, β-catenin can be activated by many growth factors, including epidermal growth factor (EGF) [5] , [6] , [7] . The increased abundance of β-catenin in the nucleus by EGF stimulation is not dependent on GSK-3β inhibition, indicating that the molecular mechanisms that regulate β-catenin stabilization and nuclear translocation are different from those of the canonical Wnt pathway [6] , [7] . Aberrant accumulation in the nucleus of β-catenin triggers upregulation of proto-oncogenes such as c-Myc and Cyclin D1 and is believed to be the basis for tumorigenesis [8] . c-Cbl has been reported as an ubiquitin E3 ligase for nuclear active β-catenin in the Wnt-on phase [9] . However, it is most likely that multiple pathways regulate the nuclear translocation and stability of β-catenin. Therefore, identifying an E3 ubiquitin ligase that generally targets nuclear β-catenin, regardless of Wnt signalling activation, would provide a broader means for targeting cancers caused by abnormal accumulation of β-catenin. Tripartite motif-containing protein 33 (TRIM33; also known as TIF1γ, RFG7, PTC7 and Ectodermin) possesses a RING domain, two B-boxes and a coiled-coil domain at the N terminus, as well as the plant homeodomain and bromodomains at the C terminus [10] . TRIM33 is a multifunctional protein that is a key regulator of embryonic and adult hematopoiesis in vertebrates [11] , facilitates efficient DNA repair [12] , regulates mitosis [13] , controls transcription elongation [14] and inhibits carcinogenesis [15] . TRIM33 has been implicated in transforming growth factor-β (TGF-β) signalling, in that it binds to phosphorylated SMAD2/3 or monoubiquitylating SMAD4 (refs 16 , 17 ). TRIM33 is also been shown to act as a tumour suppressor in hepatocellular carcinoma, human chronic myelomonocytic leukaemia and pancreatic cancer [15] , [18] , [19] . Moreover, its tumour suppression function is likely to be independent of SMAD4 (ref. 20 ), which suggests that TGF-β signalling may not be the major pathway responsible for TRIM33 abrogating tumorigenesis. However, the mechanism underlying the tumour suppression function of TRIM33 is still unknown. Here we identify TRIM33 as an E3 ubiquitin ligase for nuclear β-catenin degradation. Our data suggest that TRIM33 is a tumour suppressor that abolishes cell proliferation and tumorigenesis by degrading nuclear β-catenin. Our study has uncovered a new mechanism that controls nuclear β-catenin turnover. Its therapeutic application holds tantalizing promise in regenerative medicine. TRIM33 binds β-catenin in the nucleus To investigate a potential role for TRIM33 in regulating β-catenin stability, we first examined whether TRIM33 and β-catenin interact at the physiological level. Since TRIM33 is a nuclear protein [16] , [17] , we used nuclear extracts for co-immunoprecipitation (IP) assays. Interaction between endogenous TRIM33 and β-catenin was detected in U87 glioblastoma cells with constitutively active EGF receptor vIII (EGFRvIII) mutant and DLD-1 cells (an APC-mutant colorectal cancer cell line) ( Fig. 1a ) and with other human cells ( Supplementary Fig. 1a,b ). 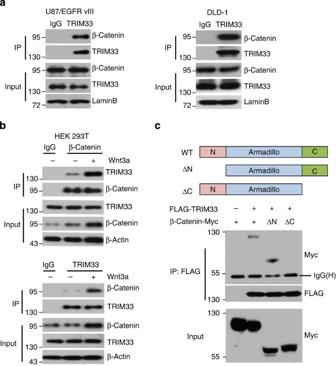Figure 1: TRIM33 binds β-catenin in the nucleus. (a) Co-IP of endogenous TRIM33 with β-catenin in U87/EGFRvIII cells (left panel) and DLD-1 cells (right panel). TRIM33 was immunoprecipitated, and the amount of TRIM33 bound to β-catenin was determined using an immunoblot with an anti-β-catenin antibody. (b) Interaction of endogenous β-catenin (top panel) and endogenous TRIM33 (bottom panel) was induced upon Wnt3a treatment. IP was performed with whole-cell lysates of HEK 293T cells pretreated with 100 ng ml−1Wnt3a. Whole-cell lysates were probed for input. The amounts of TRIM33 and β-catenin immunoprecipitated were normalized with immunoglobulin (Ig)G. (c) The C-terminal domain of β-catenin mediates the interaction of this protein with TRIM33. Top panel, schematic illustration of β-catenin. delC and delN constructs lack the C terminus and N terminus of the protein, respectively. Bottom panel, β-catenin deletion mutants were co-expressed with FLAG-TRIM33 in 293T cells in the presence of MG132. The cells were subjected to IP with a FLAG antibody followed by immunoblotting (IB) with FLAG and Myc antibodies. Whole-cell lysates were directly subjected to IB using the FLAG or Myc antibody as input. Figure 1: TRIM33 binds β-catenin in the nucleus. ( a ) Co-IP of endogenous TRIM33 with β-catenin in U87/EGFRvIII cells (left panel) and DLD-1 cells (right panel). TRIM33 was immunoprecipitated, and the amount of TRIM33 bound to β-catenin was determined using an immunoblot with an anti-β-catenin antibody. ( b ) Interaction of endogenous β-catenin (top panel) and endogenous TRIM33 (bottom panel) was induced upon Wnt3a treatment. IP was performed with whole-cell lysates of HEK 293T cells pretreated with 100 ng ml −1 Wnt3a. Whole-cell lysates were probed for input. The amounts of TRIM33 and β-catenin immunoprecipitated were normalized with immunoglobulin (Ig)G. ( c ) The C-terminal domain of β-catenin mediates the interaction of this protein with TRIM33. Top panel, schematic illustration of β-catenin. delC and delN constructs lack the C terminus and N terminus of the protein, respectively. Bottom panel, β-catenin deletion mutants were co-expressed with FLAG-TRIM33 in 293T cells in the presence of MG132. The cells were subjected to IP with a FLAG antibody followed by immunoblotting (IB) with FLAG and Myc antibodies. Whole-cell lysates were directly subjected to IB using the FLAG or Myc antibody as input. Full size image For Wnt canonical signalling, β-catenin dissociates from the APC destruction complex and translocates to the nucleus upon Wnt stimulation [3] . Indeed, we found that Wnt3a led to Wnt activation, which markedly induced the amount of endogenous TRIM33 co-immunoprecipitated with endogenous β-catenin in HEK 293T cells and vice versa ( Fig. 1b ), which suggested that TRIM33 mainly binds β-catenin in the nucleus. Experiments with β-catenin deletion mutants showed that the C terminus of β-catenin interacted with TRIM33 ( Fig. 1c ; Supplementary Fig. 1c ). Deletion of the N terminus did not change the binding affinity of TRIM33 to β-catenin, but deletion of the C terminus did ( Fig. 1c ). Thus, the C-terminal domain of β-catenin mediates the interaction of this protein with TRIM33. To examine whether the interaction between the two proteins is phosphorylation dependent, we used λ-phosphatase to treat HEK 293T cells with TRIM33 and β-catenin co-transfection. The treatment resulted in a significant dissociation of β-catenin from TRIM33, indicating that phosphorylation is necessary for TRIM33 to interact with β-catenin ( Supplementary Fig. 1d ). TRIM33 reduces the abundance of nuclear β-catenin protein Subsequently, we examined whether TRIM33 regulates the abundance of β-catenin. Overexpression of TRIM33 decreased the level of nuclear β-catenin in U87/EGFRvIII and SW480 cells (also an APC-mutant colorectal cancer cell line) ( Fig. 2a ). Conversely, depletion of TRIM33 by two independent short hairpin RNAs (shRNAs) increased the level of nuclear β-catenin in U87 cells and DLD-1 cells ( Fig. 2a ). The level also was increased by TRIM33 knockdown with small interfering RNA (siRNA) in U87/EGFRvIII cells ( Supplementary Fig. 2a ). DLD-1 cells expressed higher levels of TRIM33 than did SW480 cells, and TRIM33 expression occurred exclusively in the nucleus ( Supplementary Fig. 2b ). Moreover, immunofluorescence (IF) staining showed that when SW480 cells were transfected with FLAG-TRIM33, they expressed profoundly lower levels of endogenous β-catenin than did neighbouring untransfected cells ( Supplementary Fig. 2c ). In addition, no significant change in β-catenin messenger RNA level was detected by depletion of TRIM33, indicating that TRIM33 reduces β-catenin protein expression through post-transcriptional mechanisms ( Supplementary Fig. 2d ). 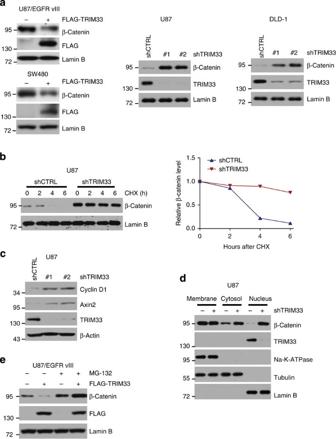Figure 2: TRIM33 reduces the abundance of nuclear β-catenin protein. (a) Left panels, U87/EGFRvIII cells or SW480 cells were transfected with an empty vector or FLAG-tagged TRIM33 expression vector. Right panels, U87 cells or DLD-1 cells were transduced using TRIM33 shRNA. Cell lysates were collected at 48 h post transfection and subjected to immunoblot analyses using the indicated antibodies. (b) TRIM33 destabilized nuclear β-catenin protein expression. Left panel, western blot of nuclear β-catenin in control-shRNA or TRIM33-shRNA U87 cells as indicated. Cells were harvested at the indicated times following inhibition of new protein synthesis by cyclohexamide (CHX). Right panel, quantitation of nuclear β-catenin normalized to the loading control and expressed relative to 0 h. (c) Cellular levels of Cyclin D1 and Axin2 in U87 cells depleted of endogenous TRIM33 were analysed by immunoblot analyses. Columns #1 and #2 indicate two independent shRNAs targeting TRIM33. (d) Cell fractions were prepared from control-shRNA or TRIM33-shRNA U87 cells. Lamin B, tubulin and Na-K-ATPase served as loading controls and cell fraction markers. (e) U87/EGFRvIII cells were transfected with or without FLAG-tagged TRIM33 treated with MG132 as indicated. Nuclear cell lysates were subjected to SDS–PAGE and immunoblot analysis using anti-β-catenin or anti-FLAG antibodies. Figure 2: TRIM33 reduces the abundance of nuclear β-catenin protein. ( a ) Left panels, U87/EGFRvIII cells or SW480 cells were transfected with an empty vector or FLAG-tagged TRIM33 expression vector. Right panels, U87 cells or DLD-1 cells were transduced using TRIM33 shRNA. Cell lysates were collected at 48 h post transfection and subjected to immunoblot analyses using the indicated antibodies. ( b ) TRIM33 destabilized nuclear β-catenin protein expression. Left panel, western blot of nuclear β-catenin in control-shRNA or TRIM33-shRNA U87 cells as indicated. Cells were harvested at the indicated times following inhibition of new protein synthesis by cyclohexamide (CHX). Right panel, quantitation of nuclear β-catenin normalized to the loading control and expressed relative to 0 h. ( c ) Cellular levels of Cyclin D1 and Axin2 in U87 cells depleted of endogenous TRIM33 were analysed by immunoblot analyses. Columns #1 and #2 indicate two independent shRNAs targeting TRIM33. ( d ) Cell fractions were prepared from control-shRNA or TRIM33-shRNA U87 cells. Lamin B, tubulin and Na-K-ATPase served as loading controls and cell fraction markers. ( e ) U87/EGFRvIII cells were transfected with or without FLAG-tagged TRIM33 treated with MG132 as indicated. Nuclear cell lysates were subjected to SDS–PAGE and immunoblot analysis using anti-β-catenin or anti-FLAG antibodies. Full size image To test whether TRIM33 regulates the stability of endogenous β-catenin, we measured the half-life of nuclear β-catenin following inhibition of new protein synthesis by cyclohexamide (CHX). The half-life was increased in TRIM33-silenced U87 cells ( Fig. 2b ). Moreover, we found that the nuclear β-catenin levels induced by Wnt3a gradually increased within 4 h and then decreased at the 8- and 16-h time points; in contrast, depletion of TRIM33 stabilized the β-catenin levels ( Supplementary Fig. 2e ). We further examined several endogenous and prototypic β-catenin target genes. Expression levels of Cyclin D1 and Axin2 proteins were increased in TRIM33-silenced U87 cells ( Fig. 2c ) and DLD-1 cells ( Supplementary Fig. 2f ). In addition, the expression of Cyclin D1 or Axin2 messenger RNA was upregulated in TRIM33-silenced U87 cells ( Supplementary Fig. 2g ). Because endogenous β-catenin exists in three distinct cellular pools [3] , we next analysed the membrane, cytosolic and nuclear quantities of endogenous β-catenin in TRIM33-silenced cell lines. Compared with the control cell lines, the membrane fraction of β-catenin was unchanged, whereas the amount of β-catenin in the cytosolic and nuclear fractions was substantially higher in the TRIM33-silenced cell lines ( Fig. 2d ). It is well known that the cytosolic and nuclear β-catenin levels are at equilibrium because β-catenin can shuttle between the cytosol and the nucleus [3] . Furthermore, TRIM33 localizes exclusively in the nucleus [16] , suggesting that TRIM33 may target only nuclear β-catenin. We thus postulated that the increased cytosolic β-catenin levels with TRIM33 suppression is directly caused by the upregulation of nuclear β-catenin levels by TRIM33 suppression. To test the idea, we generated a NES–TRIM33 construct by fusing the N terminus of FLAG-TRIM33 with a NES sequence. When NES-FLAG-TRIM33 or FLAG-TRIM33 was transfected into HEK 293T cells, the NES-FLAG-TRIM33 protein showed a mainly cytoplasmic distribution, whereas the FLAG-TRIM33 protein exhibited only nuclear accumulation in the cells ( Supplementary Fig. 3a ). Moreover, overexpression of NES-FLAG-TRIM33 did not inhibit the activity of the Wnt/β-catenin reporter ( Supplementary Fig. 3b ). Furthermore, overexpression of NES-FLAG-TRIM33 did not inhibit the cytosolic or nuclear levels of endogenous β-catenin ( Supplementary Fig. 3c ) or the EGFRvIII-driven tumour growth in vivo ( Supplementary Fig. 3d ). In contrast, overexpression of FLAG-TRIM33 in U87/EGFRvIII cells significantly suppressed the cytosolic and nuclear levels of endogenous β-catenin ( Supplementary Fig. 3c ). In addition, overexpression of FLAG-TRIM33 decreased the levels of the cytosolic and nuclear β-catenin in SW480 cells ( Supplementary Fig. 2h ). All these results indicate that cytosolic TRIM33 is deficient in degrading β-catenin, and thus that TRIM33 reduces the abundance of only nuclear β-catenin protein. To determine whether downregulation of nuclear β-catenin is mediated by the ubiquitin–proteasome pathway, we performed transient co-transfection assays in the presence or absence of the proteasome inhibitor MG132. Overexpression of TRIM33 decreased the level of nuclear β-catenin. However, MG132 blocked TRIM33-induced degradation of nuclear β-catenin in U87/EGFRvIII cells ( Fig. 2e ), suggesting that TRIM33-induced degradation of nuclear β-catenin is mediated through an ubiquitination–proteasome pathway. TRIM33-mediated destabilization is GSK-3β/β-TrCP independent In the canonical Wnt pathway, phosphorylation of β-catenin by GSK-3 followed by binding with β-TrCP results in β-catenin degradation [3] . We tested whether TRIM33-promoted β-catenin degradation requires GSK-3β or β-TrCP. Strikingly, the nuclear β-catenin levels were destabilized by overexpression of TRIM33 in GSK-3β −/− mouse embryonic fibroblasts (MEFs) ( Fig. 3a ). Because the N-terminal 47-amino-acid-spanning domain of β-catenin is targeted by the GSK-3β-regulated β-catenin degradation pathway [21] , we next determined whether the N terminus of β-catenin was dispensable for the TRIM33-repressive effect in HEK 293T cells. Data showed that the expression level of β-catenin lacking the N-terminal domain was still repressed by TRIM33 ( Fig. 3b ). Phosphorylation of the four amino-terminal serine/threonine (S33, S37, T41 and S45) residues plays a central role in β-TrCP recognition [22] . However, TRIM33 also reduced the levels of the mutant β-catenin 4SA ( Fig. 3c ). In addition, suppression of endogenous β-TrCP did not affect TRIM33-induced degradation ( Supplementary Fig. 4a ) or ubiquitination of nuclear β-catenin in U87 cells ( Supplementary Fig. 4b ). Moreover, the constitutively active β-catenin S33Y mutant, which is insensitive to GSK-3β-mediated phosphorylation and proteasomal degradation [21] , was also degraded by TRIM33 ( Fig. 3d ). All these results demonstrated that the N terminus of β-catenin is dispensable for the TRIM33-destabilizing effect ,and that TRIM33-induced β-catenin degradation does not require functional GSK-3β or β-TrCP. 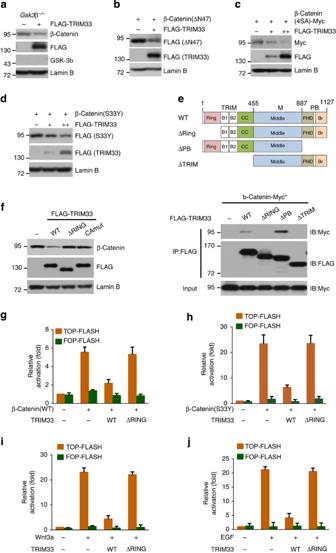Figure 3: TRIM33-mediated destabilization through the RING domain is GSK-3β or β-TrCP independent. (a) GSK-3β−/−MEFs were transfected with the constructs indicated; 48 h later, the cells were harvested and the nuclear extracts were analysed by IB. (b–d) HEK 293T cells were co-transfected with the indicated constructs; 48 h later, the cells were harvested and the nuclear extracts were analysed by IB. (e) Top panel, Diagram of TRIM33 protein domains. The N-terminal domain (TRIM) consists of a RING-finger domain, two B-box domains (B) and a coiled-coil domain (CC); the C-terminal domain consists of plant homeodomain (PHD)/bromodomain (Br) regions. Both domains are coupled by a middle region. Bottom panel, FLAG-TRIM33 and β-catenin–Myc were co-expressed in HEK 293T cells in the presence of MG132. FLAG-TRIM33 protein was immunoprecipitated using an anti-FLAG antibody. β-Catenin-bound TRIM33 protein was detected using an immunoblot with an anti-Myc antibody. Whole-cell lysates were directly subjected to IB using the anti-Myc antibody as input. (f) U87/EGFRvIII cells were transfected with the indicated plasmids, the nuclear extracts were prepared and the β-catenin level was examined. Lamin B was used as a loading control for nuclear fractions. (g) HEK 293T cells were transfected with the indicated plasmids. Transfection efficiency was normalized by co-transfection with the pRL-TK plasmid. Luciferase activity was measured 36 h after transfection by the dual-luciferase assay. Luciferase activity is shown as relative luciferase activity (RLA) compared with that in cells transfected with the control vector. (h) HEK 293T cells were transfected with the indicated plasmids. Luciferase activity was measured 36 h after transfection. (i) HEK 293T cells transfected with or without TRIM33 were transfected with TOP-FLASH or FOP-FLASH, which was followed by Wnt3a treatment for 4 h. (j) U87 cells transfected with or without TRIM33 were transfected with TOP-FLASH or FOP-FLASH, which was followed by EGF treatment for 10 h. Ing–j, each error bar indicates the variation between the means of three independent experiments. Figure 3: TRIM33-mediated destabilization through the RING domain is GSK-3β or β-TrCP independent. ( a ) GSK-3β −/− MEFs were transfected with the constructs indicated; 48 h later, the cells were harvested and the nuclear extracts were analysed by IB. ( b – d ) HEK 293T cells were co-transfected with the indicated constructs; 48 h later, the cells were harvested and the nuclear extracts were analysed by IB. ( e ) Top panel, Diagram of TRIM33 protein domains. The N-terminal domain (TRIM) consists of a RING-finger domain, two B-box domains (B) and a coiled-coil domain (CC); the C-terminal domain consists of plant homeodomain (PHD)/bromodomain (Br) regions. Both domains are coupled by a middle region. Bottom panel, FLAG-TRIM33 and β-catenin–Myc were co-expressed in HEK 293T cells in the presence of MG132. FLAG-TRIM33 protein was immunoprecipitated using an anti-FLAG antibody. β-Catenin-bound TRIM33 protein was detected using an immunoblot with an anti-Myc antibody. Whole-cell lysates were directly subjected to IB using the anti-Myc antibody as input. ( f ) U87/EGFRvIII cells were transfected with the indicated plasmids, the nuclear extracts were prepared and the β-catenin level was examined. Lamin B was used as a loading control for nuclear fractions. ( g ) HEK 293T cells were transfected with the indicated plasmids. Transfection efficiency was normalized by co-transfection with the pRL-TK plasmid. Luciferase activity was measured 36 h after transfection by the dual-luciferase assay. Luciferase activity is shown as relative luciferase activity (RLA) compared with that in cells transfected with the control vector. ( h ) HEK 293T cells were transfected with the indicated plasmids. Luciferase activity was measured 36 h after transfection. ( i ) HEK 293T cells transfected with or without TRIM33 were transfected with TOP-FLASH or FOP-FLASH, which was followed by Wnt3a treatment for 4 h. ( j ) U87 cells transfected with or without TRIM33 were transfected with TOP-FLASH or FOP-FLASH, which was followed by EGF treatment for 10 h. In g – j , each error bar indicates the variation between the means of three independent experiments. Full size image TRIM33 belongs to the TRIM protein family, which is characterized by a conserved, N-terminal tripartite motif (TRIM), a RING domain, B-box zinc-fingers and a coiled-coil region, as well as C-terminal plant homeodomain/bromodomain regions [11] . By using TRIM33 deletion mutants, we found that the interaction between TRIM33 and β-catenin was mediated by the RING domain of TRIM33 ( Fig. 3e ), indicating that this domain or its ubiquitin ligase activity is indispensable to TRIM33-induced β-catenin degradation. To follow up with this finding, we overexpressed TRIM33 without the RING domain required for interaction with β-catenin, the TRIM33 RING domain with point mutations (C125A/C128A, which destroys its E3 ubiquitin ligase activity) and wild-type (WT) TRIM33 in U87/EGFRvIII cells. WT TRIM33 decreased endogenous nuclear β-catenin levels; these levels were not decreased by either of the other mutant proteins ( Fig. 3f ), further suggesting that its ubiquitin ligase activity is critical for TRIM33-induced β-catenin degradation. The biological significance of the TRIM33–β-catenin interaction was evaluated in T-cell factor/β-catenin transcription assays. The transcriptional activities of both WT β-catenin (β-catenin WT ) and the constitutively active β-catenin S33Y were significantly blocked by the overexpression of TRIM33 ( Fig. 3g,h , respectively), confirming that TRIM33 mediated GSK-3β–independent degradation of β-catenin. Moreover, TRIM33 significantly inhibited Wnt3a- or EGF-induced β-catenin transactivation in HEK 293T cells and U87 cells ( Fig. 3i,j , respectively). However, β-TrCP overexpression in U87 cells did not change EGF-induced β-catenin transactivation ( Supplementary Fig. 4c ). All these results suggested that TRIM33-mediated Wnt-dependent and -independent β-catenin destabilization is independent of GSK-3β or β-TrCP. TRIM33 ubiquitylates nuclear β-catenin TRIM33 acts as an E3 ubiquitin ligase for several substrates [18] . Thus, we investigated whether TRIM33 could promote the ubiquitination of β-catenin. We found that TRIM33 depletion with siRNA or shRNA decreased the level of ubiquitination of nuclear β-catenin in HEK 293T cells or U87 cells ( Fig. 4a,b ; Supplementary Fig. 4d ). Conversely, TRIM33 overexpression considerably increased the level of ubiquitination of nuclear β-catenin in U87/EGFRvIII cells ( Fig. 4c ). Furthermore, TRIM33 lacking the RING domain and TRIM33 with point mutations (C125A/C128A) in the RING domain each substantially reduced the ability of TRIM33 to promote the ubiquitination of nuclear β-catenin ( Fig. 4c ), which confirmed that the RING domain or its ubiquitin ligase activity is indispensable for TRIM33-induced β-catenin degradation. 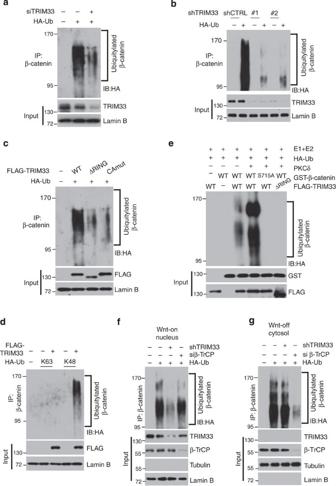Figure 4: TRIM33 ubiquitylates nuclear β-catenin. (a) HEK 293T cells with or without TRIM33 depletion by siRNA were transfected as indicated. Cells were treated with MG132 (10 μM for 4 h) prior to lysis and then subjected to anti-β-catenin IP followed by anti-HA with immunoblot analysis. (b) HEK 293T cells with or without TRIM33 depletion by shRNA were transfected as indicated. Experiments were performed as described fora. (c) Nuclear extracts of U87/EGFRvIII cells pretreated with MG132 (10 μM for 4 h) were immunoprecipitated. ΔRING, TRIM33 lacking the RING domain; CAmut, TRIM33 with point mutations (C125A/C128A) in the RING domain. (d)In vivoubiquitination assays performed in HEK 293T cells transiently transfected with HA-tagged K63-only ubiquitin or K48-only ubiquitin. (e) TRIM33 ubiquitylation of β-cateninin vitro. Purified β-catenin was subjected toin vitroubiquitylation by TRIM33 in the absence or presence of active PKCδ. β-Catenin was detected with anti-GST antibody. (f,g) U87 cells with or without TRIM33 depletion were transfected with β-TrCP siRNA or control siRNA. Cells were treated for 8 h with 100 ng ml−1Wnt3a (Wnt-on) (f) or with 100 ng DKK1 (Wnt-off) (g). Experiments were performed as described fora. Figure 4: TRIM33 ubiquitylates nuclear β-catenin. ( a ) HEK 293T cells with or without TRIM33 depletion by siRNA were transfected as indicated. Cells were treated with MG132 (10 μM for 4 h) prior to lysis and then subjected to anti-β-catenin IP followed by anti-HA with immunoblot analysis. ( b ) HEK 293T cells with or without TRIM33 depletion by shRNA were transfected as indicated. Experiments were performed as described for a . ( c ) Nuclear extracts of U87/EGFRvIII cells pretreated with MG132 (10 μM for 4 h) were immunoprecipitated. ΔRING, TRIM33 lacking the RING domain; CAmut, TRIM33 with point mutations (C125A/C128A) in the RING domain. ( d ) In vivo ubiquitination assays performed in HEK 293T cells transiently transfected with HA-tagged K63-only ubiquitin or K48-only ubiquitin. ( e ) TRIM33 ubiquitylation of β-catenin in vitro . Purified β-catenin was subjected to in vitro ubiquitylation by TRIM33 in the absence or presence of active PKCδ. β-Catenin was detected with anti-GST antibody. ( f , g ) U87 cells with or without TRIM33 depletion were transfected with β-TrCP siRNA or control siRNA. Cells were treated for 8 h with 100 ng ml −1 Wnt3a (Wnt-on) ( f ) or with 100 ng DKK1 (Wnt-off) ( g ). Experiments were performed as described for a . Full size image Lysine-48 (K48)-linked polyubiquitin chains mainly target proteins for proteasomal degradation, whereas K63-linked polyubiquitin chains are coupled to mediate nonproteolytic signals, including those that regulate subcellular localization, protein activation and protein–protein interactions [23] . By using either K63-only or K48-only ubiquitin constructs, we found that TRIM33 promotes K48 ubiquitination of β-catenin, but not K63 ubiquitination ( Fig. 4d ), suggesting that TRIM33 acts as an E3 ubiquitin ligase for β-catenin degradation. In addition, we analysed whether TRIM33 functions as a ubiquitin ligase for β-catenin in vitro and discovered that β-catenin is ubiquitylated by TRIM33 in vitro , but not by TRIM33 lacking the RING domain ( Fig. 4e ). This process was enhanced by β-catenin phosphorylation by active protein kinase Cδ (PKCδ). Therefore, TRIM33 directly polyubiquitylates β-catenin. It is well established that β-TrCP-mediated degradation of β-catenin can be a major pathway to suppressing β-catenin in the Wnt-off phase and that this degradation pathway can be inhibited in the Wnt-on phase [3] . Since TRIM33 binds and degrades the nuclear β-catenin accumulated in the Wnt-on phase, we hypothesized that TRIM33-dependent degradation of nuclear β-catenin operates mainly in this phase. To test our hypothesis, we compared the effects of depletion of β-TrCP and depletion of TRIM33 in U87 cells on the ubiquitination of cytosolic and nuclear β-catenin, as well as their half-lives in Wnt-on and Wnt-off phases. In the Wnt-on phase, the level of β-catenin ubiquitination in the nucleus was inhibited by depletion of TRIM33 ( Fig. 4f ), and the half-life of nuclear β-catenin was increased by depletion of TRIM33 ( Supplementary Fig. 5a ). However, the level of β-catenin ubiquitination and the half-life of nuclear β-catenin were not affected by depletion of β-TrCP ( Fig. 4f ; Supplementary Fig. 5a ). These results are consistent with the well-established fact that the degradation of β-catenin by β-TrCP depends on β-catenin phosphorylation at residues T41, S37 and S33 by GSK-3. In the Wnt-on phase, GSK-3 is inhibited and thus phosphorylation of β-catenin at residues T41, S37 and S33 is inhibited [22] , [24] . Moreover, it has been shown that most β-catenin in the nucleus is the non-phosphorylated (S33/S37/T41) form in the Wnt-on phase [25] . Therefore, β-TrCP-mediated degradation of nuclear β-catenin is inhibited in the Wnt-on phase. However, in our study the levels of β-catenin ubiquitination in cytosol were negligible, regardless of TRIM33 depletion or β-TrCP depletion in the Wnt-on phase ( Supplementary Fig. 5c ). In the Wnt-off phase, the level of β-catenin ubiquitination in cytosol was inhibited by depletion of β-TrCP ( Fig. 4g ), and the half-life of β-catenin in cytosol was increased by depletion of β-TrCP ( Supplementary Fig. 5b ). However, the level of β-catenin ubiquitination and the half-life of β-catenin in cytosol were not affected by depletion of TRIM33 ( Fig. 4g ; Supplementary Fig. 5b ). These results are consistent with our findings that TRIM33 is located exclusively in the nucleus ( Fig. 2d ; Supplementary Fig. 3a ) and that cytosolic NES-FLAG-TRIM33 is deficient in degrading β-catenin ( Supplementary Fig. 3 ). However, we found that the level of β-catenin ubiquitination in the nucleus was very low, regardless of TRIM33 depletion or β-TrCP depletion ( Supplementary Fig. 5d ). Collectively, the above results indicate that β-TrCP mainly ubiquitinates and degrades cytosolic β-catenin in the Wnt-off phase, whereas TRIM33 mainly targets the ubiquitination and degradation of nuclear β-catenin in the Wnt-on phase. p-β-catenin Ser715 is critical for TRIM33-induced degradation Most often, phosphorylation is necessary for a substrate to bind its E3 ligase [26] . Using β-catenin deletion mutants, we identified a binding motif in the C-terminal domain of β-catenin that was necessary to interact with TRIM33 ( Fig. 1c ). To identify the β-catenin degron sequence that determines the TRIM33 binding and subsequent ubiquitination and degradation of β-catenin, we generated several β-catenin mutants containing Ser/Thr-to-Ala mutations (S675A, T679/S680/S681-3A, T685A and S715/S718-2A) in the C-terminal domain. HEK 293T cells were transiently transfected with a TRIM33-expressing vector along with plasmids containing either β-catenin WT or each of these β-catenin mutants to test β-catenin-mediated transcriptional activity. The activities of TOP-FLASH were significantly inhibited by TRIM33 expression when cells were co-transfected with β-catenin WT or the mutants β-catenin S675A , β-catenin T679/S680/S681-3A or β-catenin T685A , but not with the mutant β-catenin S715/S718-2A ( Fig. 5a ). The results suggested that Ser715 and Ser718 located in the C-terminal domain are important for β-catenin ubiquitination and degradation. Therefore, we next examined whether Ser715 or Ser718 phosphorylation of β-catenin plays a role in TRIM33 binding. With alanine scanning mutagenesis of this region, we found that Ser715, but not Ser718, was necessary for efficient binding of β-catenin to TRIM33 ( Fig. 5b,c ). An important finding was that Ser715 was highly conserved in β-catenin orthologues ( Fig. 5d ). 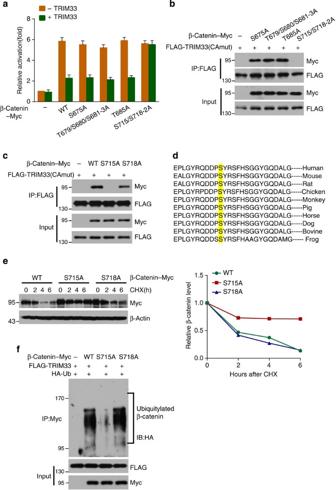Figure 5: Phosphorylation of β-catenin Ser715 is critical for TRIM33-induced β-catenin degradation. (a) HEK 293T cells were transfected with the indicated plasmids. Luciferase activity was measured 36 h after transfection. Each error bar indicates the variation between the means of three independent experiments. (b) HEK 293T cells were transfected with FLAG-tagged TRIM33 and the indicated Myc-tagged β-catenin mutants. Whole-cell lysates were immunoprecipitated with anti-FLAG antibody, and immunocomplexes were probed with antibodies against the indicated proteins. CAmut, TRIM33 with point mutations (C125A/C128A) in the RING domain. (c) HEK 293T cells were transfected with FLAG-tagged TRIM33 and the indicated Myc-tagged β-catenin mutants. Experiments were performed as described forb. (d) Alignment of the amino-acid regions containing the TRIM33-binding motif in β-catenin orthologues. (e) β-CateninS715Amutants had a longer protein half-life. Left panel, HEK 293T cells were transfected with the indicated mutants. Cells were incubated with cyclohexamide (CHX) for the indicated times, collected and analysed by IB as indicated. Right panel, the amount of β-catenin (WT or mutants) is represented relative to the amount at time 0. (f) HEK 293T cells were transfected with FLAG-TRIM33 alone or in combination with β-cateninWT–Myc or β-catenin–Myc serine substitution mutants. The transfected cells were treated with MG132 4 h prior to harvest, which was followed by IP with anti-Myc antibody. Cell lysates and the immunoprecipitates were analysed by IB with the indicated antibodies. Figure 5: Phosphorylation of β-catenin Ser715 is critical for TRIM33-induced β-catenin degradation. ( a ) HEK 293T cells were transfected with the indicated plasmids. Luciferase activity was measured 36 h after transfection. Each error bar indicates the variation between the means of three independent experiments. ( b ) HEK 293T cells were transfected with FLAG-tagged TRIM33 and the indicated Myc-tagged β-catenin mutants. Whole-cell lysates were immunoprecipitated with anti-FLAG antibody, and immunocomplexes were probed with antibodies against the indicated proteins. CAmut, TRIM33 with point mutations (C125A/C128A) in the RING domain. ( c ) HEK 293T cells were transfected with FLAG-tagged TRIM33 and the indicated Myc-tagged β-catenin mutants. Experiments were performed as described for b . ( d ) Alignment of the amino-acid regions containing the TRIM33-binding motif in β-catenin orthologues. ( e ) β-Catenin S715A mutants had a longer protein half-life. Left panel, HEK 293T cells were transfected with the indicated mutants. Cells were incubated with cyclohexamide (CHX) for the indicated times, collected and analysed by IB as indicated. Right panel, the amount of β-catenin (WT or mutants) is represented relative to the amount at time 0. ( f ) HEK 293T cells were transfected with FLAG-TRIM33 alone or in combination with β-catenin WT –Myc or β-catenin–Myc serine substitution mutants. The transfected cells were treated with MG132 4 h prior to harvest, which was followed by IP with anti-Myc antibody. Cell lysates and the immunoprecipitates were analysed by IB with the indicated antibodies. Full size image We then analysed the role of Ser715 phosphorylation in the β-catenin turnover. The β-catenin S715A mutant exhibited a longer half-life than did β-catenin WT or β-catenin S718A ( Fig. 5e ). To investigate the significance of Ser715 phosphorylation in β-catenin degradation, we assessed the ubiquitination of β-catenin WT , β-catenin S715A and β-catenin S718A . β-Catenin S715A showed decreased ubiquitination compared with β-catenin WT and β-catenin S718A in vitro ( Fig. 4e ) and in vivo ( Fig. 5f ). Consistently, in the presence of TRIM33 overexpression, the turnover rate of β-catenin WT increased compared with the control cells, but the turnover rate of β-catenin S715A did not change ( Supplementary Fig. 6 ). These findings strongly suggest that phosphorylation of β-catenin Ser715 recruits TRIM33 and that this association is critical for TRIM33-induced β-catenin degradation. PKCδ is required for the TRIM33–β-catenin interaction The discovered role of Ser715 prompted us to search for the protein kinase or kinases responsible for β-catenin phosphorylation at Ser715. Using Group-based Prediction Software (version 2.1) ( http://gps.biocuckoo.org ), we found that PKCδ is a potential serine protein kinase that phosphorylates β-catenin at Ser715. To confirm the role of PKCδ in β-catenin phosphorylation, we pretreated cells with the general PKC inhibitor bisindolylmaleimide I or the PKCα/β inhibitor Go6976. Inhibition of the general PKC, but not of PKCα/β, largely abrogated the downregulation of TRIM33-induced β-catenin transcriptional activity ( Fig. 6a ). These results implicate a role for PKC activation in β-catenin transactivation. To rule out which PKC isoform or isoforms is/are critical for TRIM33-induced β-catenin degradation, we transiently overexpressed constitutively active or kinase-dead mutants of PKCα, PKCδ and PKCε in U87/EGFRvIII cells and found that only the expression of the constitutively active mutant of PKCδ decreased nuclear β-catenin expression ( Fig. 6b ). Conversely, knockdown of PKCδ remarkably extended the protein half-life of nuclear β-catenin ( Fig. 6c ). Moreover, upon PKCδ inhibition, depletion of TRIM33 did not affect the β-catenin half-life ( Fig. 6c ) or ubiquitination ( Supplementary Fig. 7a ), indicating that PKCδ is the upstream component of TRIM33-induced β-catenin degradation. 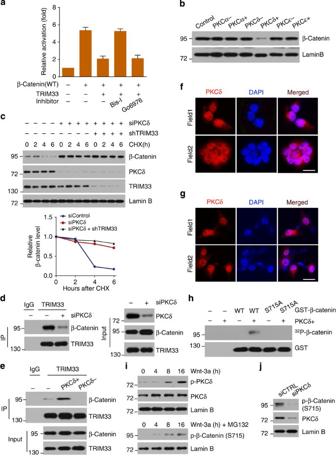Figure 6: PKCδ phosphorylates β-catenin at Ser715, promoting its association with TRIM33. (a) HEK 293T cells transiently transfected with or without TRIM33 were transfected with the indicated constructs. Cells were pretreated with Bis-I (2 mM) or Go6976 (2 mM). Each error bar indicates the variation between the means of three independent experiments. (b) U87/EGFRvIII cells were transiently transfected with constitutively active (+) or kinase-dead (−) PKC mutants. Nuclear cell lysates were collected at 48 h post transfection and subjected to immunoblot analyses using the indicated antibodies. (c) U87 cells with or without TRIM33 depletion were transfected with siRNAs targeting PKCδ or control siRNA, incubated with cyclohexamide (CHX) for the indicated times and collected and analysed. Top panel, IB results. Bottom panel, quantitation of nuclear β-catenin was normalized to the loading control and expressed relative to 0 h. (d) PKCδ silencing inhibited TRIM33–β-catenin interaction. U87/EGFRvIII cells were transfected with either a siRNA targeting PKCδ or control siRNA; 48 h post transfection, cells were collected and whole-cell lysates were immunoprecipitated and immunoblotted as indicated. (e) PKCδ stimulated the binding of TRIM33 to β-catenin. U87 cells were transiently transfected with constitutively active (+) or kinase-dead (−) PKCδ. The transfected cells were treated with MG132 4 h prior to harvest. The experiment was performed as described ind. (f,g) Localization of endogenous PKCδ in HEK 293 T (f) and U87 (g) cells. Nuclei were visualized with 4′,6-diamidino-2-phenylindole (DAPI) (blue). Scale bars, 20 μm. (h)In vitrokinase assays were performed with purified active PKCδ and purified β-catenin proteins, and analysed by autoradiography. (i) U87 cells were treated with Wnt3a (100 ng ml−1) with or without MG132 for the indicated times. IB was performed with nuclear lysates of the cells with the indicated antibody. (j) U87 cells transfected with either PKCδ siRNA targeting or control siRNA were treated with Wnt3a (100 ng ml−1) for 8 h. IB was performed with nuclear lysates of the cells with the anti-pS715-β-catenin antibody. Figure 6: PKCδ phosphorylates β-catenin at Ser715, promoting its association with TRIM33. ( a ) HEK 293T cells transiently transfected with or without TRIM33 were transfected with the indicated constructs. Cells were pretreated with Bis-I (2 mM) or Go6976 (2 mM). Each error bar indicates the variation between the means of three independent experiments. ( b ) U87/EGFRvIII cells were transiently transfected with constitutively active (+) or kinase-dead (−) PKC mutants. Nuclear cell lysates were collected at 48 h post transfection and subjected to immunoblot analyses using the indicated antibodies. ( c ) U87 cells with or without TRIM33 depletion were transfected with siRNAs targeting PKCδ or control siRNA, incubated with cyclohexamide (CHX) for the indicated times and collected and analysed. Top panel, IB results. Bottom panel, quantitation of nuclear β-catenin was normalized to the loading control and expressed relative to 0 h. ( d ) PKCδ silencing inhibited TRIM33–β-catenin interaction. U87/EGFRvIII cells were transfected with either a siRNA targeting PKCδ or control siRNA; 48 h post transfection, cells were collected and whole-cell lysates were immunoprecipitated and immunoblotted as indicated. ( e ) PKCδ stimulated the binding of TRIM33 to β-catenin. U87 cells were transiently transfected with constitutively active (+) or kinase-dead (−) PKCδ. The transfected cells were treated with MG132 4 h prior to harvest. The experiment was performed as described in d . ( f , g ) Localization of endogenous PKCδ in HEK 293 T ( f ) and U87 ( g ) cells. Nuclei were visualized with 4′,6-diamidino-2-phenylindole (DAPI) (blue). Scale bars, 20 μm. ( h ) In vitro kinase assays were performed with purified active PKCδ and purified β-catenin proteins, and analysed by autoradiography. ( i ) U87 cells were treated with Wnt3a (100 ng ml −1 ) with or without MG132 for the indicated times. IB was performed with nuclear lysates of the cells with the indicated antibody. ( j ) U87 cells transfected with either PKCδ siRNA targeting or control siRNA were treated with Wnt3a (100 ng ml −1 ) for 8 h. IB was performed with nuclear lysates of the cells with the anti-pS715-β-catenin antibody. Full size image The TRIM33-β-catenin interaction was abrogated by PKCδ depletion in U87/EGFRvIII cells ( Fig. 6d ). In addition, constitutively active PKCδ, but not kinase-dead PKCδ, enhanced the TRIM33–β-catenin interaction in U87 cells ( Fig. 6e ). These results indicate that PKCδ phosphorylation of β-catenin is required for TRIM33–β-catenin interaction. To examine the subcellular compartment in which PKCδ phosphorylates β-catenin, we conducted IF analysis. We found that most of the PKCδ was localized in the nucleus of HEK 293T cells ( Fig. 6f ) and U87 cells ( Fig. 6g ). These results suggest that PKCδ in the nucleus phosphorylates β-catenin. To examine whether PKCδ phosphorylates β-catenin directly, we conducted an in vitro kinase assay, which showed that active PKCδ was able to phosphorylate β-catenin WT , but that phosphorylation of β-catenin was completely abrogated by the S715A mutation ( Fig. 6h ). These results reveal that PKCδ directly phosphorylates β-catenin at Ser715 in vitro . Next, we investigated whether TRIM33-mediated degradation of nuclear β-catenin is a negative-feedback loop to shut down Wnt signalling upon prolonged activation. We first examined whether Wnt3a regulates PKCδ expression or activity, since TRIM33 expression level did not change upon Wnt3a stimulation. In the presence of Wnt3a, the phosphor-PKCδ level increased with prolonged treatment times (8 h and later) ( Fig. 6i ), suggesting that the PKCδ activity was changed by prolonged Wnt stimulation. We also performed Wnt treatment time-course experiments to better examine how depletion of PKCδ could affect Wnt signalling. Depletion of PKCδ stabilized the nuclear β-catenin levels induced by Wnt3a only at later time points (8 h and after) as compared with the β-catenin levels in the siControl group, despite the basal level of β-catenin at the 0 h being slightly increased in the siPKCδ group ( Supplementary Fig. 7b ). Moreover, we generated a phosphor-specific antibody against phosphor-Ser715 β-catenin. The specificity of the antibody was confirmed by the recognition of β-catenin WT protein, but not β-catenin S715A protein ( Supplementary Fig. 7c ). By using this antibody, we found a decrease in the phosphorylation status of β-catenin Ser715 with depletion of PKCδ ( Fig. 6j ), indicating that PKCδ phosphorylates β-catenin Ser715 in vivo . Moreover, β-catenin Ser715 activity gradually increased with prolonged Wnt3a treatment ( Fig. 6i ; Supplementary Fig. 3e ), indicating that the β-catenin Ser715 phosphorylation level positively correlates with the activation of Wnt signalling. These results, taken together, reveal that prolonged Wnt3a stimulation could lead to activation of PKCδ, which triggers TRIM33-dependent β-catenin degradation at later time points, serving as a negative-feedback loop for Wnt-induced β-catenin activation signalling pathways. TRIM33 abolishes tumorigenesis by destabilizing β-catenin To determine the in vivo biological significance of TRIM33 as an E3 ubiquitin ligase for β-catenin, we intracranially injected U87 cells into athymic nude mice. U87 shControl cells did not show detectable tumour formation within 2 weeks after injection ( Fig. 7a ). In contrast, depleting U87 cells of TRIM33 elicited rapid tumorigenesis, which was abrogated by knockdown of β-catenin, suggesting that TRIM33 inhibits tumorigenesis in vivo by destabilizing β-catenin. Moreover, TRIM33 overexpression abrogated EGFRvIII-driven tumour growth and it significantly inhibited β-catenin WT -, but not β-catenin S715A -, rescued brain tumour formation in U87/EGFRvIII cells ( Fig. 7b ), indicating that the β-catenin Ser715 mutation is resistant to TRIM33-induced β-catenin degradation in vivo . 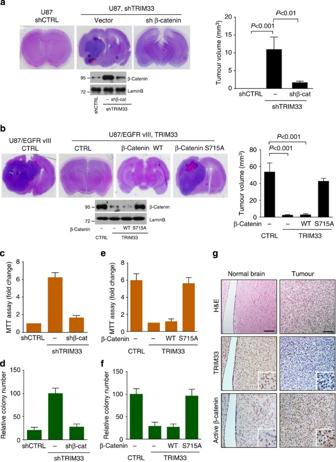Figure 7: TRIM33 abolishes tumorigenesisin vitroandin vivoby destabilizing β-catenin. (a) U87 cells with or without depleted TRIM33 and shβ-catenin were intracranially injected into athymic nude mice. After 2 weeks, the mice were sacrificed and tumour growth was examined. Left panel, top, haematoxylin and eosin (H&E)-stained coronal brain sections show representative tumour xenografts. Bottom, nuclear β-catenin levels were detected by IB analyses in these established stable cells. Right panel, Tumour volumes were measured by using length (a) and width (b) and were calculated using the equation:V=ab2/2. Data represent the results of five mice per group of two independent experiments. Error bars±s.d. Significance was determined by the Mann–WhitneyU-test. (b) U87/EGFRvIII cells with or without TRIM33 and β-catenin (WT or mutant) overexpression were intracranially injected into athymic nude mice. After 2 weeks, the mice were sacrificed and tumour growth was examined. Left panel, top, H&E-stained coronal brain sections show representative tumour xenografts. Bottom, nuclear β-catenin levels were detected by IB analyses in these established stable cells. Right panel, Tumour volumes were measured using the equation:V=ab2/2. Data represent the results of five mice per group of two independent experiments. Error bars±s.d. Significance was determined by the Mann-WhitneyU-test. (c) TRIM33-depleted U87 cells stably expressing β-catenin knockdown and their proliferation were analysed by the MTT (3-(4,5-dimethylthiazol-2-yl)-2,5-diphenyltetrazolium bromide) assay. Data are presented as mean±s.d. from three independent experiments. (d) Soft-agar assays for TRIM33-depleted U87 cells stably expressing β-catenin knockdown. Data are presented as mean±s.d. from three independent experiments. (e) TRIM33 overexpression U87/EGFRvIII cells stably expressing β-catenin (WT or mutant). Proliferation was analysed by the MTT assay. (f) Soft-agar assay for TRIM33-overexpressing U87/EGFRvIII cells stably expressing β-catenin (WT or mutant). (g) Brain tumours produced by U87/EGFRvIII cells in nude mice were processed and sectioned for immunostaining with specific antibodies against TRIM33 and active β-catenin. H&E staining revealed histopathologic features of normal mouse brain tissue and a U87/EGFRvIII tumour. Scale bars, 200 μm. Figure 7: TRIM33 abolishes tumorigenesis in vitro and in vivo by destabilizing β-catenin. ( a ) U87 cells with or without depleted TRIM33 and shβ-catenin were intracranially injected into athymic nude mice. After 2 weeks, the mice were sacrificed and tumour growth was examined. Left panel, top, haematoxylin and eosin (H&E)-stained coronal brain sections show representative tumour xenografts. Bottom, nuclear β-catenin levels were detected by IB analyses in these established stable cells. Right panel, Tumour volumes were measured by using length ( a ) and width ( b ) and were calculated using the equation: V = ab 2 /2. Data represent the results of five mice per group of two independent experiments. Error bars±s.d. Significance was determined by the Mann–Whitney U -test. ( b ) U87/EGFRvIII cells with or without TRIM33 and β-catenin (WT or mutant) overexpression were intracranially injected into athymic nude mice. After 2 weeks, the mice were sacrificed and tumour growth was examined. Left panel, top, H&E-stained coronal brain sections show representative tumour xenografts. Bottom, nuclear β-catenin levels were detected by IB analyses in these established stable cells. Right panel, Tumour volumes were measured using the equation: V = ab 2 /2. Data represent the results of five mice per group of two independent experiments. Error bars±s.d. Significance was determined by the Mann-Whitney U -test. ( c ) TRIM33-depleted U87 cells stably expressing β-catenin knockdown and their proliferation were analysed by the MTT (3-(4,5-dimethylthiazol-2-yl)-2,5-diphenyltetrazolium bromide) assay. Data are presented as mean±s.d. from three independent experiments. ( d ) Soft-agar assays for TRIM33-depleted U87 cells stably expressing β-catenin knockdown. Data are presented as mean±s.d. from three independent experiments. ( e ) TRIM33 overexpression U87/EGFRvIII cells stably expressing β-catenin (WT or mutant). Proliferation was analysed by the MTT assay. ( f ) Soft-agar assay for TRIM33-overexpressing U87/EGFRvIII cells stably expressing β-catenin (WT or mutant). ( g ) Brain tumours produced by U87/EGFRvIII cells in nude mice were processed and sectioned for immunostaining with specific antibodies against TRIM33 and active β-catenin. H&E staining revealed histopathologic features of normal mouse brain tissue and a U87/EGFRvIII tumour. Scale bars, 200 μm. Full size image With MTT (3-(4,5-dimethylthiazol-2-yl)-2,5-diphenyltetrazolium bromide) and soft-agar assays, we next examined the significance of TRIM33 as an E3 ubiquitin ligase for β-catenin in tumour cell proliferation. U87 cells with TRIM33 depletion proliferated much faster than control cells did ( Fig. 7c ). Furthermore, the ability of the shTRIM33 U87 cells to form colonies in soft agar was clearly enhanced relative to control cells, and the expression of β-catenin shRNA largely inhibited shTRIM33 U87 cell proliferation and the number of colonies ( Fig. 7d ). In addition, TRIM33 overexpression inhibited cell proliferation ( Fig. 7e ) and the number of colonies in U87/EGFRvIII cells ( Fig. 7f ); again, overexpression of TRIM33 blocked the rescuable effect of β-catenin WT , but not that of the β-catenin S715A mutant. We then used immunohistochemical (IHC) staining to evaluate the expression levels of TRIM33 and β-catenin in normal brain tissue and in brain tumours produced by U87/EGFRvIII cells or U87 stable cells in nude mice. The expression of TRIM33 was higher in normal brain tissue than in tumour tissue, whereas active β-catenin expression in the nucleus was higher in tumour tissue ( Fig. 7g ; Supplementary Fig. 8a,b ). Our observations suggested that the TRIM33 tumour suppressor function could be confirmed by IHC assessment. Level of TRIM33 inversely correlates with the β-catenin level To determine whether our findings have clinical relevance, we examined TRIM33 and β-catenin expression levels in serial sections of 40 human primary glioblastoma multiforme (GBM) specimens by IHC analyses. The levels of TRIM33 inversely correlated with the levels of active β-catenin expression in the tumours ( Fig. 8a ). Quantification of the staining showed that this correlation was statistically significant among the 40 specimens ( r =−0.528; P <0.001) ( Fig. 8b ). Moreover, among the 40 specimens, 28 included adjacent normal brain tissues, so we compared the expression level of TRIM33 in the tumours with that of the adjacent normal brain tissues. The expression level of TRIM33 in the tumours was significantly reduced compared with that in the adjacent normal brain tissues ( Fig. 8c ). Furthermore, we examined the levels of β-catenin Ser715 phosphorylation in the 40 specimens. The level of β-catenin Ser715 phosphorylation in tumours was high ( Supplementary Fig. 8c ) and inversely correlated with TRIM33 expression in tumours ( r =−0.556; P <0.001) ( Supplementary Fig. 8d ), suggesting that the accumulated phosphor-Ser715 β-catenin in GBMs was associated with the reduced TRIM33 expression. These results further support a critical role for TRIM33 in β-catenin nuclear degradation in human GBM. 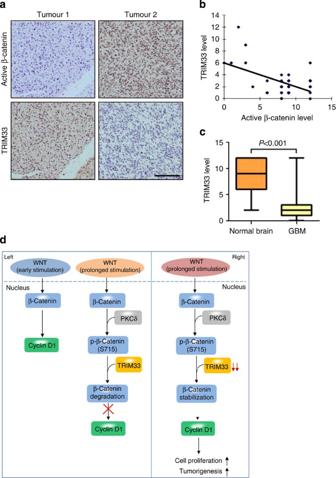Figure 8: Level of TRIM33 inversely correlates with β-catenin expression in human GBM specimens. (a) IHC staining with anti-TRIM33 and anti-active β-catenin antibodies was carried out on 40 human GBM specimens. Photographs of two representative tumours are shown. Scale bars, 200 μm. (b) Semiquantitative scoring was carried out (r=−0.528,P<0.001, Pearson correlation coefficient) with all 40 tumours. Note that some of the dots on the graphs represent more than one specimen (that is, some scores overlapped). (c) Comparison of the expression level of TRIM33 in tumours with that of the adjacent normal brain tissues in 28 specimens. Boxes indicate the interquartile range. Bars from each box extend to the largest and smallest observations.P<0.001 (Student’st-test). (d) Model for TRIM33-mediated degradation of nuclear β-catenin. Left, in cells with a level of TRIM33, which is comparable to normal cells, Wnt treatment induces the canonical Wnt/β-catenin signalling pathway activation and stabilizes β-catenin. Stabilized β-catenin that is translocated to the nucleus forms a complex with TCF/LEF-1 transcription factors, which controls the expression of many genes, such asCyclin D1. Our novel findings demonstrate that prolonged Wnt stimulation can lead to activation of PKCδ; then, phosphorylation of β-catenin at Ser715 by activated PKCδ facilitates the interaction between TRIM33 and β-catenin, which induces β-catenin degradation and hence shuts down Wnt signalling. Thus, the TRIM33-dependent β-catenin degradation serves as a negative-feedback loop to shut down Wnt signalling upon prolonged activation of the Wnt signalling. Right, in many tumour cells such as GBM cells, the level of TRIM33 is downregulated, which would result in inactivating this negative-feedback loop and hence constitutive activation of the Wnt signalling pathway to promote tumour cell proliferation and facilitate tumorigenesis. Figure 8: Level of TRIM33 inversely correlates with β-catenin expression in human GBM specimens. ( a ) IHC staining with anti-TRIM33 and anti-active β-catenin antibodies was carried out on 40 human GBM specimens. Photographs of two representative tumours are shown. Scale bars, 200 μm. ( b ) Semiquantitative scoring was carried out ( r =−0.528, P <0.001, Pearson correlation coefficient) with all 40 tumours. Note that some of the dots on the graphs represent more than one specimen (that is, some scores overlapped). ( c ) Comparison of the expression level of TRIM33 in tumours with that of the adjacent normal brain tissues in 28 specimens. Boxes indicate the interquartile range. Bars from each box extend to the largest and smallest observations. P <0.001 (Student’s t -test). ( d ) Model for TRIM33-mediated degradation of nuclear β-catenin. Left, in cells with a level of TRIM33, which is comparable to normal cells, Wnt treatment induces the canonical Wnt/β-catenin signalling pathway activation and stabilizes β-catenin. Stabilized β-catenin that is translocated to the nucleus forms a complex with TCF/LEF-1 transcription factors, which controls the expression of many genes, such as Cyclin D1 . Our novel findings demonstrate that prolonged Wnt stimulation can lead to activation of PKCδ; then, phosphorylation of β-catenin at Ser715 by activated PKCδ facilitates the interaction between TRIM33 and β-catenin, which induces β-catenin degradation and hence shuts down Wnt signalling. Thus, the TRIM33-dependent β-catenin degradation serves as a negative-feedback loop to shut down Wnt signalling upon prolonged activation of the Wnt signalling. Right, in many tumour cells such as GBM cells, the level of TRIM33 is downregulated, which would result in inactivating this negative-feedback loop and hence constitutive activation of the Wnt signalling pathway to promote tumour cell proliferation and facilitate tumorigenesis. Full size image β-Catenin stabilization increases its nuclear protein levels, and constitutive activation of β-catenin leads to tumorigenesis [3] . Phosphorylated β-catenin is specifically recognized by E3 ligase, which induces the protein’s ubiquitination and the subsequent 26S proteasomal degradation. Many E3 ubiquitin ligases that target the degradation of Wnt pathway components are known. So far, several E3 ubiquitin ligases for β-catenin degradation have been found, including β-TrCP [27] , Siah-1 (ref. 28 ), Jade-1 (ref. 29 ) and c-Cbl [9] ; all of these ligases function in a Wnt-dependent pathway. However, β-catenin can be activated by multiple pathways besides Wnt-dependent canonical signalling [5] , [6] , [7] . Searching for an E3 ligase targeting β-catenin in both Wnt-dependent and -independent pathways would provide a broader means for targeting cancers caused by aberrant activation of β-catenin. In this report, we have shown that TRIM33-mediated β-catenin destabilization is GSK-3β independent, because it can inhibit not only Wnt3a- but also EGF-induced β-catenin transactivation. Importantly, TRIM33 reduced nuclear β-catenin levels not only in colorectal cancer cell lines, in which genetic alterations in the Wnt pathway are frequently found, but also in glioblastoma cell lines, in which such genetic alterations appear to be infrequent. Moreover, TRIM33-induced β-catenin degradation did not require functional GSK-3β or β-TrCP, either of which is required for β-catenin degradation in the canonical Wnt pathway. Our discoveries that PKCδ can act as a kinase for β-catenin and phosphorylates β-catenin at Ser715, and that TRIM33 can act as an E3 ubiquitin ligase for β-catenin reveal a novel β-catenin degradation pathway ( Fig. 8d ). Our novel findings demonstrate that prolonged Wnt stimulation can lead to activation of PKCδ; then, phosphorylation of β-catenin at Ser715 by activated PKCδ facilitates the interaction between TRIM33 and β-catenin, which induce β-catenin degradation and hence shut down Wnt signalling. Therefore, our findings strongly suggest that the activation of PKCδ triggered and the TRIM33-dependent β-catenin degradation serves as a negative-feedback loop to shut down Wnt signalling upon prolonged activation. Importantly, downregulation of TRIM33, the key component in the negative-feedback loop, in GBMs would result in constitutive activation of the Wnt/β-catenin signalling pathway to promote tumour cell proliferation and facilitate tumorigenesis ( Fig. 8d ). Furthermore, PKCδ and TRIM33 in tumorigenesis have been reported to act as tumour suppressors [18] , [19] , [30] , [31] . The function of β-catenin can be regulated through Ser/Thr phosphorylation by various kinases. Previous studies have identified several Ser/Thr phosphorylation sites on β-catenin. Among them, the key N-terminal Ser and Thr residues (Ser33, Ser37, Thr41 and Ser45) have gained widespread acceptance because these sites, when phosphorylated, are essential for the ubiquitination and degradation of β-catenin [22] , [32] . In the central armadillo repeat domain of β-catenin, Wnt-induced β-catenin nuclear accumulation depends on the phosphorylation of β-catenin at Ser191 and Ser605 mediated by JNK2 kinase [33] . β-Catenin phosphorylation at Thr393 by CK2 kinase leads to proteasome resistance and increases protein stability and co-transcriptional activity [34] . AKT-mediated phosphorylation of β-catenin at Ser552 increases its nuclear accumulation by dissociating from cell–cell contacts [35] . For the C-terminal domain of β-catenin, PAK1 phosphorylates β-catenin at Ser675, which leads to more stable and transcriptionally active β-catenin [36] . However, it is unclear whether other phosphorylation sites on β-catenin regulate its degradation, especially sites not in the N-terminal residues of β-catenin containing the putative phosphodegrons. In this study, we found that the C-terminal domain of β-catenin interacted with TRIM33. We then generated several β-catenin mutants in the domain and identified that the phosphorylation of β-catenin at Ser715 was required for TRIM33-induced β-catenin ubiquitination and degradation. Thus, our results identify a novel phosphorylation site in the C terminus of β-catenin. The results also suggest that the mechanism of β-catenin degradation by TRIM33 in the nucleus is distinct from that of β-catenin degradation by the APC destruction complex in the cytoplasm. We then explored which kinase or kinases are responsible for β-catenin phosphorylation at Ser715. Using kinase-specific phosphorylation site prediction software, we found that PKCδ, which belongs to a family of serine- and threonine-specific protein kinases, is a potential serine protein kinase for β-catenin phosphorylation at this site. It is well known that the major function of PKCδ is to induce apoptosis, and for this reason it is recognized as a tumour suppressor [30] , [31] . PKCδ was recently reported to be involved in the regulation of β-catenin degradation [37] , which indicates that the role of PKCδ as a tumour suppressor is not limited to triggering apoptosis. Since aberrant nuclear accumulation of β-catenin is a widely recognized marker of poor cancer prognosis, the PKCδ tumour suppressor function may be related to β-catenin degradation. Unexpectedly, in our study, PKCδ was involved in β-catenin phosphorylation and the subsequent degradation by TRIM33. This finding elucidates the molecular mechanism of PKCδ that leads to β-catenin degradation. Some TRIM proteins (one of the subfamilies of the RING-type E3 ubiquitin ligases) function as important regulators of carcinogenesis [10] . TRIM33 was initially found to be involved in the regulation of the TGF-β pathway, where it disrupts the SMAD3–SMAD4 complex to restrict the duration of TGF-β signalling [38] . TRIM33 often is mutated, translocated or expressed at a decreased level in several human cancers, including hepatocellular cancer, pancreatic cancer and chronic myelomonocytic leukaemia [15] , [18] , [19] . Indeed, its expression was diminished in the mouse or human brain tumour tissues in our study. Although all these reports imply that TRIM33 is a tumour suppressor, the mechanism of TRIM33 tumour suppression is not clear. A recent study suggested that the role of TRIM33 as a tumour suppressor in pancreatic cancer is independent of its effect on SMAD4 (ref. 20 ), indicating that the action of TRIM33 abolishing carcinogenesis does not occur through TGF-β signalling. β-Catenin is an oncogenic protein, and its nuclear accumulation promotes tumour formation and development. In our study, TRIM33 depletion led to rapid brain tumour formation but knockdown of β-catenin inhibited the effect, suggesting that TRIM33 blocks tumour formation by destabilizing the β-catenin level. Our findings raise the possibility that the aberrant nuclear accumulation of β-catenin due to TRIM33 loss or mutation contributes to tumorigenesis. A very limited number of substrates have been reported for TRIM33 until now. Our findings also demonstrate that β-catenin is a novel substrate for TRIM33-mediated degradation. Moreover, our clinical data support the idea that TRIM33 deficiency is a mechanism for stabilizing the β-catenin substrate in human cancers. Aberrant activation of nuclear β-catenin has been implicated in a variety of human cancers and is a putative drug target [39] . β-Catenin can be activated by multiple pathways, including Wnt-dependent and -independent pathways [1] , [3] , [6] . Although the mechanisms involved in β-catenin activation are not identical across cancer types, the final result is persistent activation of β-catenin in the nucleus. Therefore, identifying an E3 ubiquitin ligase that can target nuclear β-catenin via multiple pathways would be invaluable to developing agents that can pharmacologically modulate β-catenin activity. In the past decade, various attempts have been made to identify and characterize various pharmacological inhibitors of β-catenin [39] . Our findings that TRIM33 acts as an E3 ubiquitin ligase for nuclear β-catenin will lead to new therapeutic strategies for human cancers caused by abnormal accumulation of β-catenin. Plasmids and siRNAs and reagents Human β-catenin, β-catenin mutants and human TRIM33 mutants were generated by PCR and using the QuikChange site-directed mutagenesis kit (Stratagene). The expression vectors encoding FLAG-TRIM33 and FLAG-TRIM33 CAmut were obtained from Dr Stefano Piccolo (University of Padua, Padua, Italy). FLAG-β-TrCP was obtained from Dr Peter Howley (Harvard Medical School, Boston, MA, USA). pcDNA3 S33Y β-catenin and pcDNA3 ΔN47 β-catenin were obtained from Dr Eric Fearon (University of Michigan, Ann Arbor, MI, USA). SMARTpool siRNA duplexes specific for TRIM33, PKCδ, β-TrCP and a nontargeting siRNA (siControl) were purchased from Dharmacon. Recombinant human Wnt3a, recombinant human DKK1 and recombinant human EGF were purchased from R&D Systems. PKC inhibitors bisindolylmaleimide I and Go6976 were purchased from EMD Millipore. Active PKCδ was obtained from SignalChem. Antibodies The following antibodies were from Sigma: anti-hemagglutinin (HA)-tag (H3663; 1:1,000 immunoblotting (IB)), anti-FLAG-tag (F1804; 1:1,000 IB, 2 μg IP) and anti-Myc-tag (M4439; 1:1,000 IB, 2 μg IP). The following antibodies were from Cell Signaling Technology: non-phosphor (active) β-catenin (#8814; 1:100 IHC), Axin2 (#2151; 1:1,000 IB), β-TrCP (#4394; 1:1,000 IB), PKCδ (#2058; 1:1,000 IB) and phosphor-PKCδ (Ser643/676) (#9376; 1:1,000 IB). The following antibodies were from Santa Cruz Biotechnology: β-catenin (sc-7963; 1:1,000 IB, 2 μg IP), PKCδ (sc-937; 1:100 IF), Lamin B (sc-6216; 1:1,000 IB), tubulin (sc-8035; 1:1,000 IB), normal rabbit immunoglobulin G (sc-2345; 2 μg IP), normal mouse immunoglobulin G (sc-2025; 2 μg IP), β-actin (sc-47778; 1:10,000 IB), GST (sc-138; 1:1,000 IB), GSK-3β (sc-9166; 1:1,000 IB) and Cyclin D1 (sc-753; 1:1,000 IB). The following antibodies were from Bethyl Laboratories: TRIM33 (A301-060A; 1:1,000 IB, 2 μg IP), TRIM33 (IHC-00216; 1:100 IHC). The following antibody was from BD Transduction Laboratories: β-catenin (610153; 1:100 IF). The following antibody was from Abcam: Na-K-ATPase (ab76020; 1:1,000 IB). The phosphor-Ser715 β-catenin antibody (1:1,000 IB; 1:100 IHC) was produced by Signalway Antibody (College Park, MD). Cell culture and transfection HEK 293T cells (the American Type Culture Collection, ATCC) and GSK-3β-knockout MEFs (gift from Dr James R. Woodgett, Mount Sinai Hospital, Toronto); U87 (ATCC) and U87/EGFRvIII (gift from Dr Oliver Bogler, MD Anderson Cancer Center, Houston) GBM cells; and DLD-1, SW480 and HT-29 colorectal cancer cells (ATCC) were grown in Dulbecco’s modified Eagle’s medium containing 10% fetal bovine serum (HyClone). HEK 293T cells were transfected with FuGENE HD (Roche). GSK-3β-knockout MEFs, U87, U87/EGFRvIII, DLD-1, SW480 and HT-29 cells were transfected with X-tremeGENE HP (Roche). HEK 293T, U87 and DLD-1 cells were transfected with siRNA using Lipofectamine RNAiMAX (Invitrogen). Retroviral and lentiviral generation and infection Retroviral constructs with TRIM33 -silencing constructs were co-transfected in HEK 293T packaging cells along with packaging, envelope and reverse transcriptase vectors using Lipofectamine 2000 as per the manufacturer’s instructions (Invitrogen). For TRIM33 or β-catenin (WT or mutant) ectopic expression or β-catenin silencing expression, lentiviral particles were produced using a lentivirus packaging mix (ViraPower, Invitrogen). For viral transduction, the cells were seeded at 50–60% confluence. The cells were treated overnight with the medium containing retrovirus or lentivirus harvested 48 or 72 h after transfection. Virus particles were concentrated and purified by ultra-high-speed centrifugation (25,000 g for 2 h at 4 °C). Cells were infected with retrovirus or lentivirus in the presence of 6 μg ml −1 polybrene (Sigma). Selection of stable clones was carried out using puromycin (Sigma). Subcellular fractionation For nuclear protein extraction, cells were harvested and the nuclear protein fraction was separated using the CelLytic Nuclear Extraction Kit (Sigma-Aldrich) according to the manufacturer’s recommended procedures. For experiments using membrane, cytoplasmic and nuclear protein fractions, cells were harvested and the membrane, cytoplasmic and nuclear protein fractions were separated using the Subcellular Protein Fractionation Kit for Cultured Cells (Thermo Scientific). Briefly, a cell pellet was added with cytoplasmic extraction buffer (CEB) and the tube was incubated at 4 °C for 10 min. The lysate was centrifuged at 500 g for 5 min and the supernatant was transferred (cytoplasmic extract) to a clean pre-chilled tube. The pellet was sequentially added with membrane extraction buffer and the tube was incubated at 4 °C for 10 min. The lysate was centrifuged at 3,000 g for 5 min and the supernatant was transferred (membrane extract) to a clean pre-chilled tube. The pellet (nuclear protein fraction) was collected by added IB sample buffer and boiled for 5 min. IP and IB analysis For co-IP, cells were grown in 10-cm dishes and transfected with the appropriate plasmids. Cell lysates were incubated with 2 μg of antibody on a rotator overnight at 4 °C. The protein–antibody–protein A/G-agarose complexes were prepared by adding 50 μl of protein A/G-agarose beads (Amersham Biosciences) for 1 h at 4 °C. After extensive washing with RIPA lysis buffer, the immunoprecipitated complexes were resuspended in reducing sample buffer and boiled for 10 min. After centrifugation to pellet the agarose beads, supernatants were subjected to SDS–polyacrylamide gel electrophoresis (PAGE) and IB. Full scans of IBs are presented in Supplementary Fig. 9 . IF analysis Cells were rinsed twice with phosphate-buffered saline, fixed with 4% buffered paraformaldehyde and permeabilized with 0.5% Triton X-100 for 15 min. Cells were incubated with the primary antibody overnight at 4 °C and then with the secondary antibody conjugated to rhodamine or FITC (Molecular Probes) for 1 h at room temperature. Cells were examined using a deconvolutional microscope (Zeiss). Axio Vision software from Zeiss was used to deconvolute Z-series images. Promoter reporters and dual-luciferase assay HEK 293T cells were transfected with the TOP-FLASH and FOP-FLASH reporter plasmids together with pRL-TK. Luciferase activity was measured in a 1.5-ml Eppendorf tube with the Promega Dual-Luciferases Reporter Assay kit (Promega E1980) according to manufacturer’s protocols after transfection. Relative renilla luciferase activity was normalized to firefly luciferase activity. Quantitative real-time reverse-transcription PCR Quantitative real-time reverse-transcription PCR analysis of the β-catenin gene, CTNNB1 , was performed using total RNA and the SYBR green reagent with an ABI Prism 7000HT sequence detection system. The sequences of the PCR primers were as follows: CTNNB1 forward, 5′- AGGAATGAAGGTGTGGCGACA -3′; CTNNB1 reverse, 5′- TGGCAGCCCATCAACTGGAT -3′; GAPDH forward, 5′- AATCCCATCACCATCTTCCA -3′; GAPDH reverse, 5′- TGGACTCCACGACGTACTCA -3′. The results were determined using the Comparative C t method with the housekeeping gene GAPDH as a control. In vivo ubiquitination assays HEK 293T cells were transfected with HA–ubiquitin constructs together with the indicated plasmids. Forty-eight hours after transfection, cells were harvested by sonication in ubiquitination lysis buffer (50 mM HEPES (pH 7.8), 200 mM NaCl, 5 mM EDTA, 1% NP40, 5% glycerol, 1 mM dithiothreitol, protease inhibitor cocktail (Sigma) and 250 ng ml −1 ubiquitin–aldehyde (CalBiochem)). Cell lysates were immunoprecipitated with anti-β-catenin antibody. GST-tagged protein purification GST purification of pGEX-4T-1 β-catenin (WT or mutant) constructs were performed as described previously [40] . Briefly, plasmids encoding β-catenin WT or mutant were co-transformed into Escherichia coli BL21 Rosetta cells and expressed at 18 °C for 16 h after induction with 0.2 mM isopropyl-β- D -thiogalactoside. Bacterial cell lysates were purified using Glutathione-Sepharose beads (GE Healthcare BioSciences AB). All purification steps were performed at 4 °C. In vitro ubiquitination assays FLAG-TRIM33 or its CA mutant was captured from transfected HEK 293T cell lysates by anti-FLAG agarose. After a thorough wash, the agarose was divided into aliquots. Empty anti-FLAG agarose was used as control. The in vitro ubiquitination assay was performed by incubating TRIM33-bound, mutant TRIM33-bound or control agarose at 37 °C for 1 h with E1 ubiquitin-activating enzyme UBE1, E2-conjugating enzyme UbcH5c, HA–ubiquitin and adenosine triphosphate (all from Boston Biochem) in the presence or absence of purified GST–β-catenin WT or mutant or active PKCδ. The supernatant was removed after the assay and the agarose was thoroughly washed and analysed by IB. In vitro kinase assays The kinase reactions were done by mixing purified active PKCδ and bacterially purified WT or mutant β-catenin in 20 μl of kinase assay buffer containing 10 μCi of [γ- 32 P] adenosine triphosphate, 25 mM MOPS (pH 7.2), 12.5 mM β-glycerolphosphate, 25 mM MgCl 2 , 5 mM EGTA, 2 mM EDTA, 0.25 mM dithiothreitol and 2.5 μl PKCδ lipid for 30 min at 30 °C. The reaction was stopped by the addition of sample buffer, boiled and analysed by SDS–PAGE followed by autoradiography. Pulse-chase assays U87 cells were incubated with Met- and Cys-free medium (Gibco) for 2 h, replaced with medium containing 0.2 mCi ml −1 35 S-Met (Perkin-Elmer) and incubated for 1 h. Cells were then washed three times with chase medium (Met- and Cys-free medium containing 7.5 g l −1 of methionine) and incubated with 10-fold molar excess of Cys and Met and 10% fetal calf serum in Dulbecco’s modified Eagle’s medium containing 100 ng ml −1 Wnt3a or DKK1 for 0, 4, 8 or 16 h. Cells were collected at the indicated times and β-catenin was immunoprecipitated from cell lysates using an anti-β-catenin antibody. The precipitated β-catenin was subjected to SDS–PAGE and detected with an autoradiograph. Cell proliferation and soft-agar colony formation assays For the cell proliferation assay, 5 × 10 3 cells were plated in 96-well plates. Cell growth was determined using a standard tetrazolium bromide (MTT) assay and verified by counting with trypan blue and a haemacytometer. Data represent the means±s.d. of three independent experiments. For the soft-agar assay, cells were plated at 5 × 10 4 per well using 6-well plates and were resuspended in 0.35% soft agar and layered onto 0.6% solidified agar. The soft-agar colonies were allowed to grow for 3 weeks at 37 °C. Then the cells were stained for colony visualization and counting. Experiments were carried out in triplicate. Intracranial injection All mouse experiments were approved by the Institutional Animal Care and Use Committee of The University of Texas MD Anderson Cancer Center. We intracranially injected 5 × 10 5 GBM cells with or without regulation of TRIM33 or β-catenin expression into 4-week-old female athymic nude mice (purchased from the National Cancer Institute). Five mice were injected for each group. Mice were sacrificed 2 weeks after the glioma cell injection. The brain of each mouse was harvested, fixed in 4% formaldehyde and embedded in paraffin. Tumour formation and phenotype were determined by histologic analysis of haematoxylin- and eosin-stained sections. Human or mouse tissue samples and IHC analysis Mouse tumour tissues were fixed and prepared for staining. The specimens were stained with Mayer’s haematoxylin and subsequently with eosin (Biogenex Laboratories). Afterwards, the slides were mounted using Universal Mount (Research Genetics). The tissue sections from paraffin-embedded human GBM specimens were stained with antibodies against TRIM33 and active β-catenin. IHC analyses were performed on the tissue arrays by a standard immunostaining protocol [41] . Staining was scored by two investigators blinded to the clinical data using a four-tiered system that incorporated the intensity of immunostaining and the percentage of cells that were positive. The intensity of immunostaining was scored as follows: negative, 0; weak, 1+; moderate, 2+; intense, 3+. For tumours that showed heterogeneous staining, the predominant pattern was taken into account for scoring. The percentage of positive cells was divided into five grades (percentage scores): <10% (0), 10–25% (1), 26–50% (2), 51–75% (3) and >75% (4). The use of human brain tumour specimens was approved by the institutional review board at The University of Texas MD Anderson Cancer Center, and written informed consent was obtained from the patients for the use of clinical specimens for research. Statistical analysis The significance of the data from patient specimens was determined by the Pearson correlation coefficient test. The significance of the in vitro data and in vivo data between experimental groups was determined by Student’s t -test or Mann–Whitney U -test. P <0.05 was considered to be significant. How to cite this article: Xue, J. et al . Tumour suppressor TRIM33 targets nuclear β-catenin degradation. Nat. Commun. 6:6156 doi: 10.1038/ncomms7156 (2015).